Comprehensive study of the spin-charge interplay in antiferromagnetic La2−xSrxCuO4 The origin of the pseudogap and its relationship with superconductivity in the cuprates remains vague. In particular, the interplay between the pseudogap and magnetism is mysterious. Here we investigate the newly discovered nodal gap in hole-doped cuprates using a combination of three experimental techniques applied to one, custom made, single crystal. The crystal is an antiferromagnetic La 2− x Sr x CuO 4 with x =1.92%. We perform angle-resolved photoemission spectroscopy measurements as a function of temperature and find: quasi-particle peaks, Fermi surface, anti-nodal gap and below 45 K a nodal gap. Muon spin rotation measurements ensure that the sample is indeed antiferromagnetic and that the doping is close, but below, the spin-glass phase boundary. We also perform elastic neutron scattering measurements and determine the thermal evolution of the commensurate and incommensurate magnetic order, where we find that a nodal gap opens well below the commensurate ordering at 140 K, and close to the incommensurate spin density wave ordering temperature of 30 K. Recent low-temperature angle-resolved photoemission spectroscopy (ARPES) experiments on the underdoped cuprate superconductors indicate the presence of a fully gapped Fermi surface (FS) [1] , [2] , [3] , [4] ; even in the antiferromagnetic phase [5] . The natural candidates for opening such a gap are charge or spin density waves (SDW). Out of all hole-doped cuprates, La 2− x Sr x CuO 4 (LSCO) is the most promising material for exploring whether a SDW is indeed responsible for this gap. LSCO single crystals with large size allow for magnetic measurements such as muon spin rotation (μSR) and neutron diffraction (ND), simultaneously with ARPES. The magnetic probes can characterize the SDW while ARPES explores the gap. However, the region of the phase diagram where the magnetic properties are clearly exposed is different from the region where the band dispersion is visible. On the one hand, long-range magnetic order disappears as doping approaches 2% from below, hindering our ability to perform ND. On the other hand, LSCO becomes insulating at low temperature as the doping approaches 2% from above, thus restricting ARPES. In fact, ARPES data for LSCO with doping lower than 3% are rare and missing the quasiparticle peaks in the energy distribution curves (EDCs) [2] , [6] . The main problem is the high resistivity of extremely underdoped samples, which is detrimental to ARPES due to charging effects. Nevertheless, the resistivity of LSCO as a function of temperature, at 2% doping, has a broad minimum around 100 K [7] . This minimum insures that resistivity is finite even at lower temperatures and opens a window for both experiments. By preparing a series of LSCO single crystals with ~0.2–0.3% doping steps around 2%, we manage to find one to which all techniques apply. This allows us to explore the cross-talk between the magnetic and electronic properties of the material. We find that the charge excitation are impartial to the commensurate spin order. However, the nodal gap opens at a temperature very close to the one where an incommensurate SDW sets in. The small temperature mismatch is assigned to experimental sensitivity. The magnetic order The series of samples are first characterized by μSR. In Fig. 1 , we show the μSR frequency as a function of temperature for all crystals. In samples with doping equal to or less than 2%, the oscillation starts at temperatures on the order of 100 K. At 2%, there is a sharp transition from the antiferromagnetic long-range order to the spin-glass state where the same oscillations appear only at temperatures on the order of 10 K (refs 8 , 9 ). More details of the μSR characterization of the samples are given below and in the Methods section. 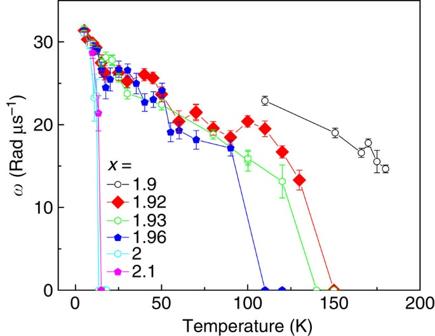Figure 1: μSR frequency as a function of temperature. μSR frequency as a function of temperature for LSCO single crystals with differentxvalues. Atx=2%, there is a clear transition from an antiferromagnetic to a spin-glass ground states. The data in the rest of this paper are measured on thex=1.92% sample, which is in the antiferromangetic phase. The error bars were determined from the data fitting procedure described in the Methods section. We perform the ND and ARPES measurements on a sample with x =1.92% (red rhombuses) that is antiferromagnetic with a Néel temperature T N ≃ 140 K. Figure 1: μSR frequency as a function of temperature. μSR frequency as a function of temperature for LSCO single crystals with different x values. At x =2%, there is a clear transition from an antiferromagnetic to a spin-glass ground states. The data in the rest of this paper are measured on the x =1.92% sample, which is in the antiferromangetic phase. The error bars were determined from the data fitting procedure described in the Methods section. 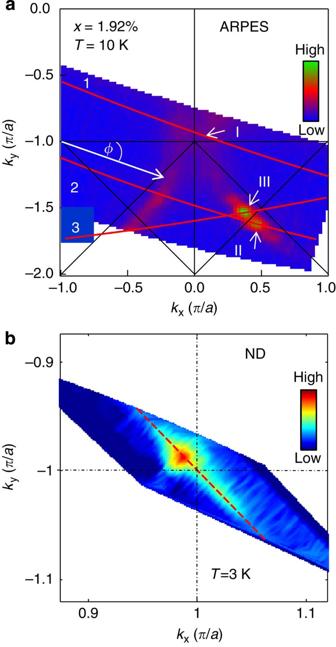Figure 2: The Fermi surface and incommensurate magnetic order in LSCO with 1.92% doping. (a) Low-energy ARPES data in the second Brillouin zone. The red lines 1 and 2 show cuts on which data were collected. Line 3 is the cut on which temperature dependence data are presented inFig. 3. Point I, II and III mark points where EDCs are extracted. The intensity is centred in the diagonal region. (b) ND measurements at 3 K in a small region around a magnetic reciprocal lattice vector showing a strong and feeble incommensurate peaks. The dashed red line depicts the measurements scan direction. Full size image The FS Figure 2a shows the ARPES intensity map near the Fermi level ( E F ) in the second Brillouin zone, measured along cuts parallel to cut 1 and 2 shown in the figure. The high intensities represent the underlying FS and has the morphology of the FS in more doped LSCO [10] and other cuprates. Most of the intensity is centred around the zone diagonal on the (0, −2 π / a ) to ( π / a , − π / a ) line. This suggests the presence of gapped electronic excitations in the off-diagonal (0, − π / a ) region. Similar results were obtained at a higher doping level of x =3−8% (ref. 4 ). Figure 2: The Fermi surface and incommensurate magnetic order in LSCO with 1.92% doping. ( a ) Low-energy ARPES data in the second Brillouin zone. The red lines 1 and 2 show cuts on which data were collected. Line 3 is the cut on which temperature dependence data are presented in Fig. 3 . Point I, II and III mark points where EDCs are extracted. The intensity is centred in the diagonal region. ( b ) ND measurements at 3 K in a small region around a magnetic reciprocal lattice vector showing a strong and feeble incommensurate peaks. The dashed red line depicts the measurements scan direction. Full size image The magnetic structure Figure 2b depicts ND for the same sample at 3 K. The scans are performed along the red line, in a narrow range in the reciprocal lattice space centred around the (1, −1) point, in the standard tetragonal ARPES units of π / a . In fact, the scanned area of the ND experiment in k-space is only a small fraction of the scanned area of the ARPES. A clear breaking of the fourfold symmetry is observed in this figure. In addition, two incommensurate peaks are present in the centre of the figure: one is clearly observed as a red spot, and the other is weak and will be demonstrated below. Such incommensurate peaks occur when, on top of the main magnetic order, the system develops spin modulations (stripes) running in diagonal to the bond directions (diagonal stripes). The stripes and commensurate scattering observed in our sample are in agreement with previous reports for low-doping LSCO [11] , [12] , and are discussed further below. The gap In Fig. 3a–h , we show the temperature dependence of ARPES data in the vicinity of point III along cut 3 in Fig. 2a . All spectra are divided by resolution broadened Fermi-Dirac distribution at the nominal temperature. Data analysis by the Lucy–Richardson deconvolution method [13] is discussed in the Methods section. At high temperatures ( T >50 K), the dispersive peak crosses E F as clearly seen in Fig. 3a . In contrast, at low temperatures ( T <45 K), there is a gap in the electronic spectra, that is, the peak position at k F remains below E F . A similar gap exists in LSCO up to 8% doping [4] , in LBCO at 4% (ref. 2 ), in the electron doped compound [1] , in Bi2212 (ref. 3) [3] and La-Bi2201 (ref. 5) [5] . It also exsists in simulations where inhomogeneous SDW and superconductivity coexist [14] or Coulomb disorder effects are present [15] . EDCs extracted from Fig. 3a–h , at k F given by point III of Fig. 2a , are plotted in Fig. 3i . The solid lines are guides to the eye. At temperatures above 45 K, the peak is at E F . However, below this temperature the peaks are clearly below E F , indicating the presence of a gap. 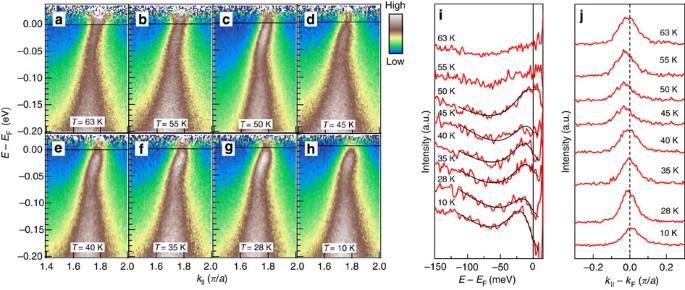Figure 3: Temperature dependent ARPES data. (a–h) ARPES spectra along a cut given by line 3 inFig. 1. The spectra are divided by resolution broadened Fermi-Dirac distribution. At highT,the spectrum crosses the Fermi energy. At lowT,it does not. (i) EDCs at the Fermi momentum of point III inFig. 1bfor different temperatures. The solid lines are guides to the eye. At 10 K, the peak is clearly below the Fermi energy. Δ(T) is presented inFig. 4c. (j) MDC atEFas a function of temperature showing thatkFin the diagonal region is temperature independent. Figure 3: Temperature dependent ARPES data. ( a – h ) ARPES spectra along a cut given by line 3 in Fig. 1 . The spectra are divided by resolution broadened Fermi-Dirac distribution. At high T, the spectrum crosses the Fermi energy. At low T, it does not. ( i ) EDCs at the Fermi momentum of point III in Fig. 1b for different temperatures. The solid lines are guides to the eye. At 10 K, the peak is clearly below the Fermi energy. Δ( T ) is presented in Fig. 4c . ( j ) MDC at E F as a function of temperature showing that k F in the diagonal region is temperature independent. Full size image An important aspect of these EDCs is the fact that at all low temperatures, E F is not in the middle of the gap, namely, the intensity of the spectra immediately above E F is lower than at E F . This could be an analysis artifact due to division by the resolution broadened Fermi-Dirac function [13] or indicate that the particle-hole symmetry is broken. Particle-hole asymmetry towards the diagonal region in the non-superconducting phase [16] , and in the off-diagonal region [17] , was found previously. However, it is very difficult to distinguish between the two options in our sample with extremely low carrier concentration. Another parameter relevant for understanding the mechanism by which the nodal gap opens is the temperature dependence of k F . This is explored by extracting the momentum dispersion curve at E F from Fig. 3a–h , as presented in Fig. 3j . The peak position fluctuates somewhat around a constant value as the temperature is lowered, indicating that k F =0.63( π / a ) along the diagonal is temperature independent. Therefore, the high-intensity curves in Fig. 2b represents the FS. The evolution of the gap around the FS is shown in Fig. 4a,b for 10 and 100 K. The spectra marked I and II in Fig. 4a are EDCs at the k F of points I and II in Fig. 2a . The spectra in between correspond to k F between points I and II. EDCs shown in Fig. 4b are from similar point along the FS. In the off-diagonal region, there is no spectral weight at E F for both temperatures, indicating that the anti-nodal gap opens at a temperature higher than 100 K. In the diagonal region, there is high spectral weight at 100 K, but not at 10 K. Thus at 100 K, we observe a Fermi arc [18] , while at 10 K, a gap appears all around the FS. 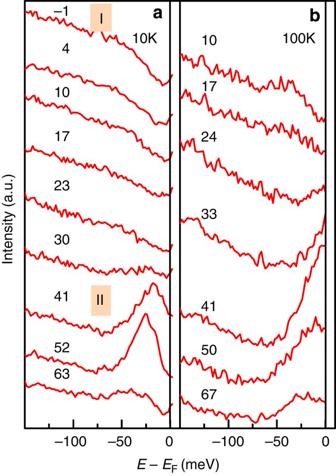Figure 4: Angular-dependent ARPES data. (a) EDCs at differentkFalong the FS in two different temperatures. The Fermi surface angleφis indicated above each EDC. Spectra I and II are taken at the k of point I and II inFig. 1bthat are defined by the crossing point between the red lines 1 and 2 and the FS. The other EDCs are from the crossing points in between. At 10 K, a gap is observed all around the FS. Δ(φ) is presented in the inset ofFig. 5c. (b) Similar EDCs at 100 K. In this case, a gap is observed only in the off-diagonal region. Figure 4: Angular-dependent ARPES data. ( a ) EDCs at different k F along the FS in two different temperatures. The Fermi surface angle φ is indicated above each EDC. Spectra I and II are taken at the k of point I and II in Fig. 1b that are defined by the crossing point between the red lines 1 and 2 and the FS. The other EDCs are from the crossing points in between. At 10 K, a gap is observed all around the FS. Δ( φ ) is presented in the inset of Fig. 5c . ( b ) Similar EDCs at 100 K. In this case, a gap is observed only in the off-diagonal region. Full size image Summary of parameters Finally, in Fig. 5 , we present a summary of parameters extracted from all three techniques. 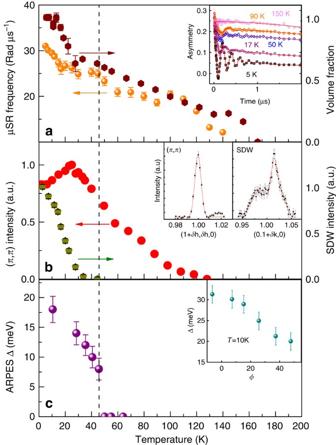Figure 5: Experimental parameters from all three techniques. (a) Muon rotation frequency and the magnetic volume fraction of the sample as a function of temperature taken from a fit to a three Lorentzian model (see Methods section). The inset shows raw data and the fit quality for thex=1.92% sample. (b) Commensurate and incommensurate ND intensity. The SDW inset is the intensity versuskalong the neutron scattering cut inFig. 2cshowing the strong and feeble incommensurate peaks. The (π,π) inset shows the commensurate peak. (c) ARPES nodal gap Δ atkF, as obtained from the peaks inFig. 3i, versus temperature. The inset shows the angular dependence of the gap Δ(φ). The error bars were determined from the experimental resolution. Figure 5a shows the temperature dependence of the muon rotation frequency and magnetic volume fraction. The inset represents a fit of a three-component model, with one frequency, to the μSR data at different temperatures. More details are available in the methods section. The magnetic parameters grow upon cooling, saturate between 50 and 25 K, and grow again at lower temperatures. The temperature T F =25 K was associated with hole freezing into one dimensional domain walls [8] , [9] , [19] . The restriction of the charge motion below T F must be intimately related to the opening of the nodal gap. Figure 5: Experimental parameters from all three techniques. ( a ) Muon rotation frequency and the magnetic volume fraction of the sample as a function of temperature taken from a fit to a three Lorentzian model (see Methods section). The inset shows raw data and the fit quality for the x =1.92% sample. ( b ) Commensurate and incommensurate ND intensity. The SDW inset is the intensity versus k along the neutron scattering cut in Fig. 2c showing the strong and feeble incommensurate peaks. The ( π , π ) inset shows the commensurate peak. ( c ) ARPES nodal gap Δ at k F , as obtained from the peaks in Fig. 3i , versus temperature. The inset shows the angular dependence of the gap Δ( φ ). The error bars were determined from the experimental resolution. Full size image Figure 5b shows the commensurate and the incommensurate scattering intensity. The insets show two raw data sets. The first is a scan along (0,1+ δk ,0) (in orthorhombic units), which is the red diagonal line in Fig. 2b . This scan is sensitive to the incommensurate fluctuations and show two asymmetric peaks. The second scan is along (1+ δh ,1,0) and detects only the commensurate order as a single peak. As the temperature is raised, the incommensurate intensity decreases until it disappears at T F =30 K. The commensurate intensity peaks at 25 K , just when the muon oscillation changes its behaviour, and vanishes at T N =130 K. Our ND temperature dependence results, shape of the peaks and incommensurability parameter (in tetragonal units) δ =0.027( π / a ) are in good agreement with previously reported data [12] . While the ND data are well understood in terms of a spiral ground state [20] , its relation to the gap is still mysterious, since the nesting condition is not fulfilled in our sample. The nodal gaps at k F , Δ, are determined from the peak in the EDCs of Fig. 3i and presented in Fig. 5c as a function of temperature. Very similar gap values are found using the Lucy–Richardson deconvolution method, shown in Fig. 6 (ref. 13 ). The gap opens at 45 K. The major observations in this figure are: (I) the nodal gap opens when the commensurate moment is about half its full value. (II) With temperature decreasing, the nodal gap first opens when the incommensurate moment is barely or not detectable. 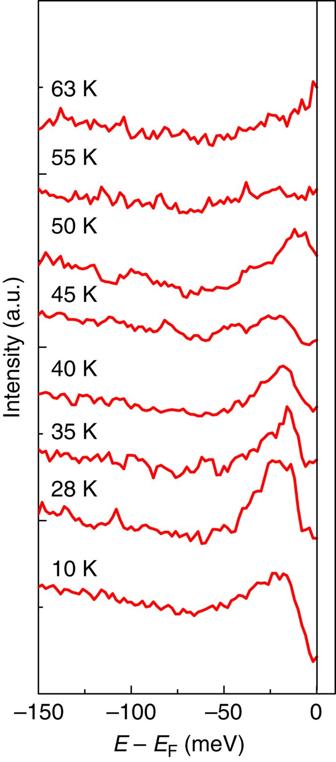Figure 6: The Lucy–Richardson method. The same data as inFig. 3ibut analysed using the Lucy–Richardson deconvolution method13. Figure 6: The Lucy–Richardson method. The same data as in Fig. 3i but analysed using the Lucy–Richardson deconvolution method [13] . Full size image The temperature mismatch between the opening of the nodal gap and appearance of the incommensurate peaks could be real, but most likely is an artifact. We determined the ARPES gap from the quasi-particle peaks. An alternative is to use the leading edge as the measure of the gap. The leading edge crosses the Fermi energy at a lower temperature than the peak. Therefore, the leading edge criteria would make the temperature mismatch smaller. In addition, the ND require both periodic and frozen magnetic moments on a time scale determined by the instrument resolution. ARPES is sensitive to shorter time scales than ND. Hence, lower temperature are required for ND to pick up the incommensurate signal than for ARPES to detect the gap. This experimental time scale difference between techniques is an alternative explanation to the temperature mismatch. The angular dependence of the gaps is presented in the inset of Fig. 5c ; the angle φ is defined in Fig. 2a . When a peak is absent, the gap is taken from the change of slope in the EDCs. Δ( φ ) is in agreement with previous measurements for 3–8% dopings [4] . On the basis of weak coupling theory, Berg et al . [21] argued that the commensurate part of the SDW can open a nodal gap only if the moment is larger than a critical value. However, the opening of the gap will be accompanied by a shift in k F . The effect of the incommensurate part of the SDW depends on the properties of time reversal followed by translation symmetry, which can be broken or unbroken. In the unbroken case, a nodal gap will open when the perturbation exceeds a critical value. Both these options do not agree with our data. In the broken symmetry case, a nodal gap can open for arbitrarily small perturbation with no impact on k F . This option is in agreement with our measurements and bares important information on the symmetries of the ground state. Another possibility is that the gap is of the superconducting type, which maintains particle-hole symmetry and keeps k F fixed. This option would mean that the cuprates have a superconducting gap in the antiferromagnetic phase. In conclusion, we detect a nodal gap in the antiferromagnetic phase of LSCO. The gap opens well below T N and very close to the temperature where incommensurate SDW is detected. This finding puts strong restrictions on the origin of the nodal gap. μSR The experiment was carried out at PSI on the GPS beam line. We fit the muon polarization as a function of time to where ω is the muon rotation angular frequency, V m stands for the magnetic volume fraction, p is the amplitude of the rotating signal resulting from the angle between the muon spin and the internal field, D , R 1 and R 2 are relaxation rates, b 1 and b 2 are stretching exponents, and P Bg is the background polarization from muon that missed the sample. We could fit the data well with b 1 =0.5 and b 2 =1 for most of the temperatures. Between T =25 to 50 K, we allowed freedom in their values to achieve an optimal fit. ARPES The experiment was done at the Swiss Light Source in PSI. The samples were mounted on a specialized holder, as described in Mansson et al . [22] , with silver glue to improve electrical conductivity. The Fermi level and resolution were determined from the polycrystalline copper sample holder. The samples were cleaved in situ at T =10 K under a ultrahigh vacuum better than 6 × 10 −11 Torr. Circularly polarized light with hv =55 eV was used. The spectra were acquired with a VG Scienta R4000 electron analyser. Charging tests have been carried out by varying the photon flux. No charging was found. In addition, after performing the high temperature measurements, the sample was cooled again and the results at 10 K were reproducible. We examined the surface with LEED at each temperature and no surface degeneration or reconstruction was found during the measurements. It should be pointed out that in ARPES, the incoming light warms the surface, and there could be a few degrees difference between the sample surface temperature and the temperature of the cold finger which we quote in the paper. EDCs obtained by Lucy–Richardson deconvolution method are depicted in Fig. 6 . Neutron diffraction The ND experiments was carried out at Paul Scherrer Institute (SINQ, PSI) on the RITA-II beam line. The crystal was mounted on an aluminium sample holder with the crystallographic ĉ -axis perpendicular to the neutron beam; that is, (1,0,0)–(0,1,0) scattering plane. The beam collimation was set to 80′-40′-80′. A beryllium filter was placed before the analyser to remove higher order neutrons. The instrument consisted of a nine-blade pyrolytic graphite analysers. The diffraction studies were performed with 4.04 Å (5 meV) neutrons, using all the blades in order to create a 2D intensity plot. The sample was aligned in such a manner that the area of interest (commensurate and incommensurate magnetism) was measured in the centre blade. The incommensurate part was measured in a (0,1+ δq ,0) scan to avoid the commensurate contribution. The high temperature data weres subtracted to remove the leftover λ /2 contribution form the (0,2,0) structural Bragg peak. For the commensurate part, the measurement was performed with a scan direction (1+ δq , δq ,0) to avoid the incommensurate contribution. How to cite this article : Drachuck, G. et al . Comprehensive study of the spin-charge interplay in antiferromagnetic La 2− x Sr x CuO 4 . Nat. Commun. 5:3390 doi: 10.1038/ncomms4390 (2014).